Inhibition of miR-146a prevents enterovirus-induced death by restoring the production of type I interferon There are no antivirals or vaccines available to treat Enterovirus 71 (EV71) infections. Although the type I interferon response, elicited upon virus infection, is critical to establishing host antiviral innate immunity, EV71 fails to induce this response efficiently. Here we provide new insights into potential anti-EV71 therapy by showing that neutralization of EV71-induced miR-146a prevents death in mice by restarting the production of type I interferon. EV71 infection upregulates miR-146a, which targets IRAK1 and TRAF6 involved in TLR signalling and type I interferon production. We further identify AP1 as being responsible for the EV71-induced expression of miR-146a. Surprisingly, knocking out miR-146a or neutralizing virus-induced miR-146a by specific antagomiR restores expressions of IRAK1 and TRAF6, augments IFNβ production, inhibits viral propagation and improves survival in the mouse model. Our results suggest that enterovirus-induced miR-146a facilitates viral pathogenesis by suppressing IFN production and provide a clue to developing preventive and therapeutic strategies for enterovirus infections. Enterovirus 71 (EV71), which was first identified in California in 1969, has become a newly emerging life-threatening pathogen, particularly in the Asia-Pacific region, since 1997. Severe EV71 outbreaks with dozens of fatalities were first noted in Malaysia in 1997 and in Taiwan in 1998. Fatal cases have been reported in Japan (1997), Singapore (2000), China (2008) and Korea (2009), and cases with severe neurological disease have also been identified in Western Australia [1] , [2] , [3] , [4] , [5] . However, there is no effective therapy or vaccine for EV71 infection [4] . EV71 can infect humans through fecal–oral route and spread to the central nervous system (CNS) including spinal cord, parietal and frontal cerebral lobes, midbrain, pons, medulla and cerebellum [6] . Infection with EV71 results in typical hand-foot-and-mouth disease, encephalomyelitis, pulmonary oedema, poliomyelitis-like paralysis or even neurological and psychiatric complications [6] , [7] , [8] , [9] . EV71 infection can result in acute pulmonary edema, with the sudden onset of tachycardia, tachypnea, cyanosis and shock several hours to days after onset of CNS involvement, and in most such cases, the patient will die hours later [6] , [10] . Even though some EV71-infected individuals with pulmonary edema survive under modern intensive care, most of the survivors have long-term neurological sequelae or impaired cognitive function. Therefore, an effective antiviral therapy is necessary to reduce the case-fatality rate and the long-term sequelae. Generally, virus-associated molecules are recognized by host pattern-recognition receptors and activate endosomal toll-like receptor (TLR) signalling to produce type I interferons (IFNs) [11] , [12] . The resulting IFNs can establish antiviral machinery in virus-infected individuals by inducing interferon-stimulated genes, promoting the proliferation of memory T cells, stimulating IFNγ production and activating dendritic cells and natural killer cells [13] , [14] , [15] , [16] . Intriguingly, EV71 does not effectively stimulate infected hosts to produce type I IFNs as observed in humans or in animal models [17] , [18] . However, type I IFN treatment could improve and even cure EV71 infections [17] , [19] , [20] , [21] , [22] , [23] . These findings imply that the sequelae and mortality might be reduced if the production of type I IFNs can be normally induced during EV71 infection. Virus infections can alter host gene expression profiles, including miRNAs, contributing to viral propagation and pathogenesis [24] . Our previous study showed that EV71 upregulates miR-141 expression through induction of EGR1. The virus can suppress host eukaryotic initiation factor 4E, shutting down cap-dependent translation and augmenting virus propagation [25] . In addition, miR-122 is able to stabilize HCV genomic RNA, while suppressing miR-122 by a locked nucleic acid-modified oligonucleotide (LNA) attenuated HCV replication in a chimpanzee model [26] , [27] . A phase IIa clinical trial conducted to assess the safety and efficacy of an LNA-based miR-122 inhibitor looks particularly compelling because of its lack of any known adverse effects [28] . This exciting example suggests that miRNAs may serve as promising targets for antiviral therapy. Herein, we hypothesize that host miRNAs might be involved in EV71 pathogenesis through suppression of type I IFN induction and could act as candidates for developing antiviral therapy. Targets of virus-induced miR-146a Previously, we have reported that the host miRNA expression profile was altered in EV71 infection assayed in RD cells [25] . Besides miR-141, miR-146a, another EV71-induced microRNA was selected for further investigation in this study due to its regulatory activity in TLR signalling and IFN production ( Supplementary Fig. 1a ). 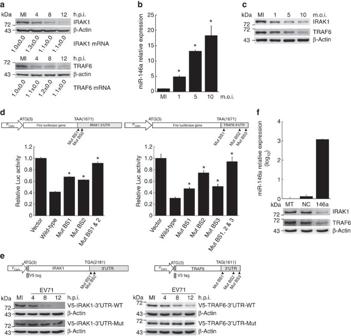Figure 1: IRAK1 and TRAF6 are the targets of EV71-induced miR-146a. (a) EV71 infection suppressed IRAK1 and TRAF6 expressions in protein level. (b,c) miR-146a induction and IRAK1 and TRAF6 suppressions were dose dependent. *P-value <0.05, Student’st-test, as compared with mock infection. (d) The effect of miR-146a on the luciferase reporter vectors harbouring wild-type or mutant 3′UTRs (n=4). *P-value <0.05, Student’st-test, as compared with wild-type 3′UTR. (e) EV71 suppressed the expressions of V5-IRAK1 and V5-TRAF6 with wild-type 3′UTRs. (f) The effect of ectopic miR-146a on endogenous expression of IRAK1 and TRAF6. RD cells were transfected with the miR-146a overexpressing vector or negative control and assayed for IRAK1 and TRAF6, and miR-146a by western blot and real-time RT–PCR (n=3), respectively. MI, mock infection; MT, mock transfection; NC, negative control. All data presented are mean±s.d. Seventy-nine potential miR-146a targets were predicted by TargetCombo [29] ( Supplementary Table 1 ). Among these targets, IRAK1 and TRAF6, two key elements involved in TLR signalling and IFN production, have already been reported as miR-146a targets that contribute to the proinflammation response and tumorigenesis in various tissues and physiological situations [30] , [31] , [32] . To determine whether IRAK1 and TRAF6 were affected by EV71 infection, RD cells derived from human rhabdomyosarcoma were infected with EV71, and IRAK1 and TRAF6 expressions were detected at different time points post infection. The expressions of both proteins were suppressed, but mRNA expressions were not ( Fig. 1a ). Taken together, these results indicate that miR-146a could be induced by EV71 infection and might target IRAK1 and TRAF6. Moreover, we performed dose response experiments to evaluate whether the induction of miR-146a and suppression of IRAK1 and TRAF6 were dose dependent or not, and the results indicated under EV71 infection, they were ( Fig. 1b,c ). We also checked whether live virus was essential for the two phenomena to occur. Supplementary Fig. 1c revealed that live virus did obviously induce miR-146a expression and further suppress IRAK1 and TRAF6, while heat-killed virus did not alter the expression levels of miR-146a, IRAK1 and TRAF6. The evidence indicated that live virus was essential for initiation of the miR-146a cascade. However, the exact miR-146a binding sites (BS) of IRAK1 and TRAF6 have not yet been thoroughly validated, nor has the suppressive activity associated with each BS been evaluated. Hence, we used PicTar ( http://www.pictar.org/ ) and RNA22 ( http://www.cbcsrv.watson.ibm.com/rna22.html ) [33] , [34] to predict the potential miR-146a BS within the 3′UTR of IRAK1 and TRAF6 ( Supplementary Fig. 1b ). Next, 3′UTRs of IRAK1 and TRAF6 with or without 4-base mutations in the predicted miR-146a BS were constructed into miRNA reporter vectors. The reporter assays demonstrated that all of the predicted miR-146a BS in the 3′UTRs of IRAK1 and TRAF6 are essential for miR-146a-mediated suppression. For vectors with all the mutated BS, miR-146a had lost almost all suppressive activity ( Fig. 1d and Supplementary Fig. 2 ). We further elucidated whether the suppression of IRAK1 and TRAF6 in EV71 infection is miR-146a dependent. To do so, V5-IRAK1-3′UTR-WT, V5-IRAK1-3′UTR-Mut (combining all the mutant BS), V5-TRAF6-3′UTR-WT and V5-TRAF6-3′UTR-Mut stably expressing cells were established and infected with EV71, after which the protein expressions of V5-IRAK1 and V5-TRAF6 were measured at indicated time points. V5-IRAK1 and V5-TRAF6 were markedly suppressed in cases of wild-type 3′UTR, but not in cases of mutant 3′UTR ( Fig. 1e ). Figure 1f shows that the ectopic expression of miR-146a can directly suppress the protein expression of the endogenous IRAK1 and TRAF6. We demonstrated that EV71 infection induces miR-146a, which targets IRAK1 and TRAF6 and suppresses their protein expressions. However, the underlying mechanism by which miR-146a is upregulated in EV71 infection remains unclear. Figure 1: IRAK1 and TRAF6 are the targets of EV71-induced miR-146a. ( a ) EV71 infection suppressed IRAK1 and TRAF6 expressions in protein level. ( b , c ) miR-146a induction and IRAK1 and TRAF6 suppressions were dose dependent. * P -value <0.05, Student’s t -test, as compared with mock infection. ( d ) The effect of miR-146a on the luciferase reporter vectors harbouring wild-type or mutant 3′UTRs ( n =4). * P -value <0.05, Student’s t -test, as compared with wild-type 3′UTR. ( e ) EV71 suppressed the expressions of V5-IRAK1 and V5-TRAF6 with wild-type 3′UTRs. ( f ) The effect of ectopic miR-146a on endogenous expression of IRAK1 and TRAF6. RD cells were transfected with the miR-146a overexpressing vector or negative control and assayed for IRAK1 and TRAF6, and miR-146a by western blot and real-time RT–PCR ( n =3), respectively. MI, mock infection; MT, mock transfection; NC, negative control. All data presented are mean±s.d. Full size image AP1 upregulates miR-146a expression Transcription factors have been demonstrated to bind onto miRNA regulatory elements and further govern miRNA expression [25] , [35] . The miR-146a promoter region was defined in 2006 by Taganov et al . [32] , and the promoter region was used to seek potential BS of the transcriptional factor(s). To determine the transcription factor(s) responsible for regulation of virus-induced miR-146a, we first predicted the potential BS for the transcription factors within the miR-146a promoter region with TRANSFAC, JASPAR and Promo software and then intersected the results with EV71-altered transcription factors in RD cells assayed by microarrays [25] , [36] , [37] , [38] . 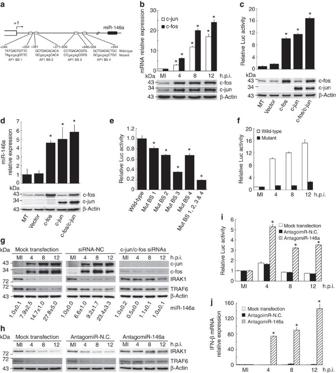Figure 2: Regulation of miR-146a and the effect of EV71-induced miR-146a on interferon production. (a) Schematic organization of miR-146a. AP1 (c-jun/c-fos) BS were predicted by intersection of TRANSFAC, PROMO and JASPAR software. (b) AP1 was upregulated by EV71 infection (n=3). MI, mock infection. *P-value <0.05 compared with mock infection. (c,d) c-jun and c-fos enhance the promoter activity and expression of miR-146a. RD cells were transfected with the c-jun or c-fos overexpressing vector and assayed for promoter activity (n=4) (c) and miR-146a expression (n=3) (d). MT, mock transfection. *P-value <0.05 as compared with vector control. (e) Determination of AP1 BS within miR-146a promoter. AP1 core sequence mutants are indicated ina. The transcriptional activities of miR-146a mutant promoters were determined in the presence of AP1 (n=4). *P<0.05 as compared with the wild-type control. (f) EV71 activated miR-146a promoter harbouring a natural context but not a mutant one (n=4). (g) Silencing of AP1 decreased virus-induced miR-146a expression and restored IRAK1 and TRAF6. (h) Suppression of IRAK1 and TRAF6 was restored by antagomiR-146a. (i) Inhibition of IFNβ promoter activity was attenuated by antagomiR-146a. IFNβ promoter was constructed and assayed by promoter assays (n=4). *P-value <0.05 as compared with antagomiR-N.C. (j) AntagomiR-146a eliminated the suppression of IFNβ expression in EV71 infection. IFNβ expressions were determined by real-time RT–PCR (n=3). MI, mock infection. *P-value <0.05 as compared with antagomiR-N.C. All data presented are mean±s.d. and allP-values are calculated by Student’st-test. AP1 (c-jun/c-fos) was the only candidate identified in the intersection ( Supplementary Table 2a,b ). Four potential AP1 BS were predicted within the miR-146a promoter region ( Fig. 2a and Supplementary Table 2c ). The AP1 (c-jun/c-fos) expressions at both the mRNA and protein levels were significantly increased during EV71 infection ( Fig. 2b and Supplementary Fig. 3a ). The miR-146a promoter region was constructed into a luciferase reporter vector and assayed in the presence of c-jun and c-fos. Enforced expression of c-jun and c-fos enhanced the transcriptional activity of miR-146a promoter as well as the expression of the endogenous miR-146a ( Fig. 2c,d ). To further verify the direct activation activity of AP1 on miR-146a expression, we generated constructs containing individual mutations for each potential AP1 BS within the miR-146a promoter region ( Fig. 2a and Supplementary Table 2c ) and determined the importance of each AP1 BS by reporter assays. The third AP1 BS was more potent than the others on the transcriptional regulation of miR-146a. However, all four BSs contributed to miR-146a upregulation, for the luciferase activity of the vector with all four mutant AP1 BSs was the most greatly suppressed ( Fig. 2e ). Moreover, the wild-type or each of the four miR-146a promoter constructs with AP1 BS mutant was transfected into host cells before virus infection to evaluate the contribution of AP1 to miR-146a promoter activity. The AP1 BS mutation almost completely abolished the induction activity of the miR-146a promoter caused by EV71 infection ( Fig. 2f ). This data indicated that AP1 is the key transcription factor contributing to EV71-induced upregulation of miR-146a. Previous studies have reported that RelA, RelB and p50 could regulate miR-146a expression and suggested that miR-146a expression was NF-κB-dependent [32] , [39] , [40] , [41] , [42] . To verify whether NF-κB is involved in EV71-induced miR-146a upregulation, NF-κB translocation and NF-κB activity were examined in EV71-infected RD cells and assayed by NF-κB immunoblot and NF-κB regulatory element assays. The results showed that NF-κB was not translocated into the nucleus and that NF-κB signalling was suppressed in EV71 infection ( Supplementary Fig. 3b,c ). We also examined the NF-κB status in EV71-infected Caco-2 and THP-1 cells. The results indicated that NF-κB was not translocated into the nucleus in either Caco-2 or THP-1 cells during EV71 infection ( Supplementary Fig. 5d,g ). These results suggested that NF-κB was not involved in the miR-146a induction in EV71 infection. We suggest that virus-induced AP1 could upregulate miR-146a and thereby cause IRAK1 and TRAF6 suppression. To address this issue, c-jun and c-fos siRNAs (5 pM for each siRNA) were introduced into host cells before virus infection, and IRAK1, TRAF6 and miR-146a were assayed by western blot and real-time RT–PCR. miR-146a expression was inhibited and IRAK1 and TRAF6 were restored in the presence of c-jun and c-fos siRNAs ( Fig. 2g ). On the other hand, host cells were treated with JNK inhibitor (SP600125), which inhibits the activation of JNK pathway and further decreases c-jun and c-fos expression [43] , [44] before virus infection. AP1 expression was inhibited by JNK inhibitor, accompanied with suppression of miR-146a and restoration of IRAK1 and TRAF6, as in the cases of c-jun and c-fos siRNAs ( Supplementary Fig. 4 ). IRAK1 and TRAF6 are the two key components in the signalling pathway of type I IFN production [11] , [45] . To explore whether the recovery of IRAK1 and TRAF6 by silencing of miR-146a could restore the production of IFNs in EV71 infection, antagomiR-146a (5 pM) was transfected into host cells before virus infection. We found that IRAK1 and TRAF6 recovered remarkably ( Fig. 2h ), and IFNβ promoter activity was restored at 4 hours post infection (h.p.i.) as compared with negative controls or mock transfection ( Fig. 2i ). The IFNβ mRNA expression was increased dramatically in antagomiR-146a transfectants as assayed by real-time RT–PCR ( Fig. 2j ). Neutralization of miR-146a rescued IRAK1 and TRAF6 expressions and in turn restored IFN production in EV71-infected cells. Figure 2: Regulation of miR-146a and the effect of EV71-induced miR-146a on interferon production. ( a ) Schematic organization of miR-146a. AP1 (c-jun/c-fos) BS were predicted by intersection of TRANSFAC, PROMO and JASPAR software. ( b ) AP1 was upregulated by EV71 infection ( n =3). MI, mock infection. * P -value <0.05 compared with mock infection. ( c , d ) c-jun and c-fos enhance the promoter activity and expression of miR-146a. RD cells were transfected with the c-jun or c-fos overexpressing vector and assayed for promoter activity ( n =4) ( c ) and miR-146a expression ( n =3) ( d ). MT, mock transfection. * P -value <0.05 as compared with vector control. ( e ) Determination of AP1 BS within miR-146a promoter. AP1 core sequence mutants are indicated in a . The transcriptional activities of miR-146a mutant promoters were determined in the presence of AP1 ( n =4). * P <0.05 as compared with the wild-type control. ( f ) EV71 activated miR-146a promoter harbouring a natural context but not a mutant one ( n =4). ( g ) Silencing of AP1 decreased virus-induced miR-146a expression and restored IRAK1 and TRAF6. ( h ) Suppression of IRAK1 and TRAF6 was restored by antagomiR-146a. ( i ) Inhibition of IFNβ promoter activity was attenuated by antagomiR-146a. IFNβ promoter was constructed and assayed by promoter assays ( n =4). * P -value <0.05 as compared with antagomiR-N.C. ( j ) AntagomiR-146a eliminated the suppression of IFNβ expression in EV71 infection. IFNβ expressions were determined by real-time RT–PCR ( n =3). MI, mock infection. * P -value <0.05 as compared with antagomiR-N.C. All data presented are mean±s.d. and all P -values are calculated by Student’s t -test. Full size image miR-146a signalling cascade is ubiquitous To explore whether this miR-146a signalling cascade exists in another important EV71 primarily targeted organ, the intestine, Caco-2 cells, derived from colon adenocarcinoma, were substituted for RD cells to investigate the miR-146a regulation. Caco-2 cells were infected with EV71 and analysed for the expression of c-jun, c-fos, miR-146a, IRAK1 and TRAF6 at indicated h.p.i. EV71 infection induced the expression of miR-146a and suppressed IRAK1 and TRAF6 ( Fig. 3a,b ). AP1 was upregulated in mRNA and protein levels starting at 12 h.p.i. ( Fig. 3c ). Suppression of IRAK1 and TRAF6 could also be restored in the presence of antagomiR-146a (5 pM) as compared with negative controls ( Fig. 3d ). This evidence implied that AP1-mediated miR-146a induction and IRAK1 and TRAF6 suppression are ubiquitous regulations occurring in different EV71-infected cell types. Again, miR-146a induction and IRAK1 and TRAF6 suppression were all regulated in a dose-dependent manner ( Supplementary Fig. 5a,b ). Live EV71 is essential for the induction of miR-146a and suppression of IRAK1 and TRAF6 ( Supplementary Fig. 5c ). THP-1 cells, a human monocyte-like cell line, were also used to evaluate the miR-146a cascade. AP1 could be induced in EV71-infected THP-1 cells, and the miR-146a expression was further upregulated ( Supplementary Fig. 5e,f ). We then investigated whether the upregulation of miR-146a is a common characteristic in enterovirus infections. The expression of miR-146a was measured in RD cells infected with two other enteroviruses, poliovirus type 3 (PV3, Sabin strain) and coxsackievirus B3 (CVB3). As shown in Fig. 3e,f,g , CVB3 and PV3 infections induced miR-146a expression and AP1 upregulation as well as the suppression of IRAK1 and TRAF6. Having demonstrated the importance of miR-146a in type I IFN production in vitro , we thus further evaluated the role of miR-146a in vivo , especially focusing on IFN production and pathogenesis. 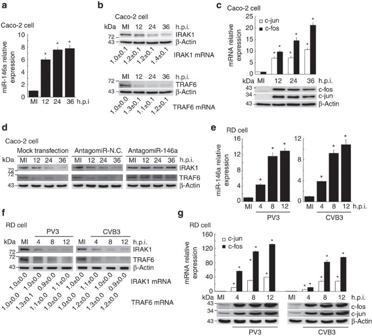Figure 3: Induction of miR-146a is an ubiquitous phenomenon across cell types and enterovirus genus. (a–c) EV71 infection induced miR-146a expression (n=3) (a), suppressed IRAK1 and TRAF6 expressions (b) and enhanced AP1 expression (n=3) (c) in Caco-2 cells. MI, mock infection. (d) AntagomiR-146a restored EV71-induced suppression of TRAF6 and IRAK1 in Caco-2 cells. Caco-2 cells were transfected with antagomiR-146a or antagomiR-N.C. before virus infection. (e–g) PV3 and CVB3 infections induced miR-146a expression (n=3) (e), suppressed IRAK1 and TRAF6 expressions (f) and enhanced AP1 expression (n=3) (g) in RD cells. *P-value <0.05, Student’st-test, as compared with mock infection. Figure 3: Induction of miR-146a is an ubiquitous phenomenon across cell types and enterovirus genus. ( a – c ) EV71 infection induced miR-146a expression ( n =3) ( a ), suppressed IRAK1 and TRAF6 expressions ( b ) and enhanced AP1 expression ( n =3) ( c ) in Caco-2 cells. MI, mock infection. ( d ) AntagomiR-146a restored EV71-induced suppression of TRAF6 and IRAK1 in Caco-2 cells. Caco-2 cells were transfected with antagomiR-146a or antagomiR-N.C. before virus infection. ( e – g ) PV3 and CVB3 infections induced miR-146a expression ( n =3) ( e ), suppressed IRAK1 and TRAF6 expressions ( f ) and enhanced AP1 expression ( n =3) ( g ) in RD cells. * P -value <0.05, Student’s t -test, as compared with mock infection. Full size image miR-146a is critical for EV71 pathogenesis in vivo To characterize the role of miR-146a in EV71 infection in vivo , we have generated a mouse-adapted EV71 strain (designated as mEV71 thereafter) for establishing an EV71 infection mouse model due to the low- or non-infectivity of human EV71 in mice [9] . We first examined the miR-146a signalling cascade in mouse embryonic fibroblast (MEF) cells. Because the sequences of mus and homo miR-146a are identical, we speculated that mus miR-146a might bind onto mus IRAK1 and TRAF6 3′UTRs and suppress their expressions. There are three potential BS within mus IRAK1 3′UTR but only two within mus TRAF6 3′UTR ( Fig. 4c and Supplementary Table 3 ). We predicted the potential targets for mus miR-146a involved in immune response through the pathway analysis of mus miR-146a target genes, which was performed with MetaCore software. 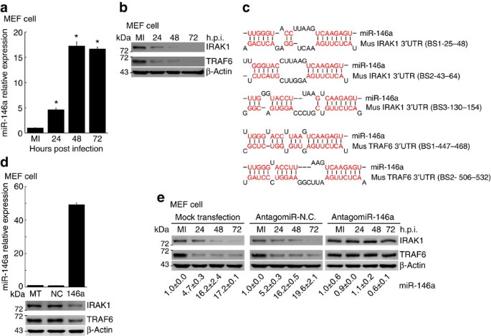Figure 4: IRAK1 and TRAF6 are the targets of mus miR-146a. (a) miR-146a was induced in mEV71 infection. MEF cells were infected with mEV71, followed by quantification of miR-146a using real-time RT–PCR (n=3). MI, mock infection. *P-value <0.05 as compared with mock infection. (b) mEV71 infection suppressed IRAK1 and TRAF6 expressions in protein level in MEF cells. (c) Predicted mus miR-146a BSs within mus IRAK1 and TRAF6 3′UTRs (the first nucleotide following the stop codon was designated as +1). (d) The effect of the ectopic miR-146a on the endogenous IRAK1 and TRAF6. MEF cells were transfected with the miR-146a overexpressing vector or negative control and assayed for IRAK1 and TRAF6 and for miR-146a by western blot and real-time RT–PCR, respectively (n=3). MT, mock transfection; NC, negative control. (e) AntagomiR-146a restored mEV71-induced suppression of TRAF6 and IRAK1 in MEF cells. MEF cells were transfected with antagomiR-146a or antagomiR-NC followed by mEV71 infection. All data presented are mean±s.d. and allP-values are calculated by Student’st-test. Besides IRAK1 and TRAF6, two immune-related targets were predicted, CD28 and SMAD4 ( Supplementary Table 4 ). MEF cells were infected with mEV71, and the expression levels of miR-146a and IRAK1 and TRAF6 were detected by real-time RT–PCR and western blot, respectively. The results suggested that mEV71 could induce the expression of miR-146a and the suppression of IRAK1 and TRAF6 ( Fig. 4a,b ). Figure 4d indicates that the ectopic expression of miR-146a could directly suppress the endogenous IRAK1 and TRAF6 in MEF cells. Furthermore, to evaluate whether the suppressions of IRAK1 and TRAF6 were indeed caused by miR-146a, antagomiR-146a were transfected into MEF cells, followed by mEV71 infection. The results showed that IRAK1 and TRAF6 were restored remarkably as compared with mock transfection or antagomiR-NC ( Fig. 4e ). Based on these results, it was clear that the miR-146a signalling cascade existed in MEF cells. For in vivo mEV71 infection assays, the optimal viral doses were determined by using different plaque-forming units (PFUs). The 10-day survival rate of mice infected with 1 × 10 8 and 2 × 10 8 PFUs of mEV71 through the natural oral route were 60 and 20%, respectively, so these doses were selected for further experiments ( Supplementary Fig. 6a ). The miR-146a expressions of the major organs in miR-146a knockout mice were checked by real-time RT–PCR. However, the miR-146a expressions of the organs assayed were varied in wild-type mice but were undetectable in miR-146a −/− mice ( Supplementary Fig. 7 ). Both wild-type and miR-146a −/− mice were fed with two doses of mEV71 as indicated and the clinical symptoms were recorded daily. The 10-day survival rates of wild-type mice infected with 2 × 10 8 and 1 × 10 8 PFUs were 27 and 54%, respectively. Surprisingly, the survival rates of miR-146a −/− mice infected with 2 × 10 8 and 1 × 10 8 PFUs significantly increased to 92 and 93% at 10 days post infection (d.p.i.) (Student’s t -test, P =0.0013 and 0.0212, respectively) ( Fig. 5a ). These results implied that the knockout of miR-146a could improve survival in EV71 infection. Next, we found that the mEV71-infected mice displayed rear limb paralysis, but mock-infected mice did not ( Fig. 5b and Supplementary Movies 1 and 2 ). The muscle tissues of mEV71-infected mice presented severe necrotizing myositis as compared with mock-infected mice, assayed by hematoxylin and eosin staining ( Fig. 5b ). Interestingly, pulmonary edema was found in mEV71-infected mice ( Fig. 5b ). We further addressed whether necrotizing myositis was directly associated with virus infection. EV71 was obviously detected in muscles with necrotizing myositis by immunohistochemistry staining ( Fig. 5b , lower panel). A previous study demonstrated that a high viral load in tissue was accompanied by severe signs of illness and high mortality [46] . Due to the dramatic difference in mortality between wild-type and miR-146a −/− mice, we measured EV71 titres in all major organs at 1 h.p.i. and 3 d.p.i. by plaque assays. It was reasonable that higher titers of EV71 were detected in the gastrointestinal tract (stomach, intestine and rectum) of both wild-type and miR-146a −/− mice at 1 h.p.i. due to EV71 infection through oral administration. Three days later, the viral loads were much higher in the major EV71 susceptible organs [4] , [8] , [9] , [10] , [47] , [48] (intestine, muscle, brain, spinal cord and lung) of the wild-type mice than in those of mice with miR-146a −/− ( Fig. 5c ). Moreover, the presence of EV71 in the blood of wild-type mice, but not miR-146a −/− mice, at 3 d.p.i. indicated that viremia occurred only in wild-type mice and that miR-146a knockdown restricted the spread of EV71 [49] , [50] , [51] . These data implied that a systemic EV71 infection occurred in wild-type mice but not in miR-146a −/− mice. Taken together, these data at least partially explained why miR-146a −/− mice were more resistant to EV71 infection and why high viral loads could cause high mortality, as reported previously [46] . Figure 4: IRAK1 and TRAF6 are the targets of mus miR-146a. ( a ) miR-146a was induced in mEV71 infection. MEF cells were infected with mEV71, followed by quantification of miR-146a using real-time RT–PCR ( n =3). MI, mock infection. * P -value <0.05 as compared with mock infection. ( b ) mEV71 infection suppressed IRAK1 and TRAF6 expressions in protein level in MEF cells. ( c ) Predicted mus miR-146a BSs within mus IRAK1 and TRAF6 3′UTRs (the first nucleotide following the stop codon was designated as +1). ( d ) The effect of the ectopic miR-146a on the endogenous IRAK1 and TRAF6. MEF cells were transfected with the miR-146a overexpressing vector or negative control and assayed for IRAK1 and TRAF6 and for miR-146a by western blot and real-time RT–PCR, respectively ( n =3). MT, mock transfection; NC, negative control. ( e ) AntagomiR-146a restored mEV71-induced suppression of TRAF6 and IRAK1 in MEF cells. MEF cells were transfected with antagomiR-146a or antagomiR-NC followed by mEV71 infection. All data presented are mean±s.d. and all P -values are calculated by Student’s t -test. 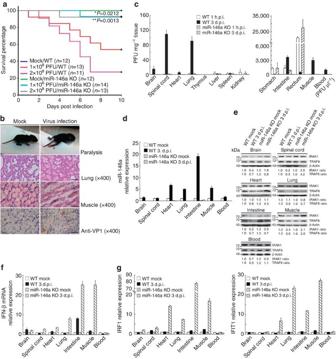Figure 5: Mortality and suppression of IFN production are dramatically improved in mEV71-infected miR-146−/−mice. (a) miR-146a−/−mice displayed significantly high survival rates. miR-146a−/−mice or wild-type mice were infected with mEV71 and monitored daily for determination of survival rate. * represents the comparison between the 1 × 108PFU/miR-146a KO group and the 1 × 108PFU/WT group; ** represents the comparison between the 2 × 108PFU/miR-146a KO group and the 2 × 108PFU/WT group. (b) Representative clinical signs of paralysis and histological examinations in mEV71-infected mice. Magnifications, × 400; scale bar represented 200 μm. (c) Virus propagations were restricted in miR-146a−/−mice. Viral loads in indicated tissues were measured by plaque assay (n=4). The expressions of miR-146a (n=3) (d), IRAK1 and TRAF6 (e), IFNβ (n=3) (f) and IRF1 and IFIT1 (n=3) (g) in mEV71-infected wild-type or miR-146a−/−mice (mouse tissue samples pooling,n=4). The Kaplan–Meier method was used to estimate overall survival and the Log-rank test was performed to test the difference between survival curves. Full size image Figure 5: Mortality and suppression of IFN production are dramatically improved in mEV71-infected miR-146 −/− mice. ( a ) miR-146a −/− mice displayed significantly high survival rates. miR-146a −/− mice or wild-type mice were infected with mEV71 and monitored daily for determination of survival rate. * represents the comparison between the 1 × 10 8 PFU/miR-146a KO group and the 1 × 10 8 PFU/WT group; ** represents the comparison between the 2 × 10 8 PFU/miR-146a KO group and the 2 × 10 8 PFU/WT group. ( b ) Representative clinical signs of paralysis and histological examinations in mEV71-infected mice. Magnifications, × 400; scale bar represented 200 μm. ( c ) Virus propagations were restricted in miR-146a −/− mice. Viral loads in indicated tissues were measured by plaque assay ( n =4). The expressions of miR-146a ( n =3) ( d ), IRAK1 and TRAF6 ( e ), IFNβ ( n =3) ( f ) and IRF1 and IFIT1 ( n =3) ( g ) in mEV71-infected wild-type or miR-146a −/− mice (mouse tissue samples pooling, n =4). The Kaplan–Meier method was used to estimate overall survival and the Log-rank test was performed to test the difference between survival curves. Full size image To further verify miR-146a-mediated signal transduction, the expression levels of miR-146a, IRAK1, TRAF6 and IFNβ were assayed. miR-146a expressions were greatly increased in heart, lung, intestine and muscle, but less increased in brain, spinal cord and blood in wild-type mice upon EV71 infection ( Fig. 5d ). A reciprocal correlation was found between miR-146a expression and the expressions of its target genes, IRAK1 and TRAF6; that is, higher miR-146a expression was associated with lower expression of IRAK1 and TRAF6 in wild-type mice ( Fig. 5e ). In addition, IFNβ production was also reciprocally correlated to miR-146a expression, especially in heart, lung, intestine and muscle ( Fig. 5f ). Two IFN-stimulated genes (ISGs), interferon regulatory factor 1 (IRF1) and interferon-induced protein with tetratricopeptide repeats 1 (IFIT1) were selected, and the expression levels were detected in all assayed groups to strengthen the claims. The results indicated that these two ISGs could be upregulated in miR-146a − / − mice infected with mEV71 as compared with a mock control group, especially in heart, lung, intestine and muscle. However, there were no significant differences in comparisons between wild-type mice infected with mEV71 and the mock control group ( Fig. 5g ). In the case of miR-146a −/− mice, we could not detect any increased miR-146a expression in any of the assayed organs. Consistently, there were no obvious decreases in the expression of IRAK1 and TRAF6 or inhibition of IFNβ, IRF1 and IFIT1 relative to the mock control group ( Fig. 5e,f,g ). Furthermore, body weight decreased much more in wild-type mice infected with 2 × 10 8 PFUs than in the EV71-infected miR-146a −/− mouse group or mock groups ( Supplementary Fig. 8a ). These data clearly indicate that miR-146a governs EV71 pathogenesis, including viral propagation, IFN blockage, clinical illness and even mortality. LNA antagomiR-146a may serve as a potential anti-EV71 drug The inhibition of miR-122 is a very promising discovery in terms of decreasing HCV viral loads in vivo and suggests a new therapeutic strategy for controlling virus infection by neutralization of the host miRNAs induced in virus infection [26] , [27] , [52] , [53] , [54] , [55] . Even though the importance of miR-146a in EV71 pathogenesis was clearly elucidated by using the miR-146a −/− mouse model, the therapeutic potential of miR-146a silencing should be practically evaluated in the EV71 infection mouse model. LNA antagomiR-146a, a designed LNA, was first injected intraperitoneally for evaluation of the potential adverse effects caused by the LNA antagomiRs (1.2 mg kg −1 ). The blood chemistry report showed no significant pathological changes after the injection of LNA antagomiR-NC or LNA antagomiR-146a ( Supplementary Table 5 ). After guaranteeing the safety of LNA antagomiRs, we next introduced LNA antagomiR-146a into wild-type mice before or after virus infection as indicated and monitored the clinical symptoms of the mice daily. Injection of LNA antagomiR-146a (1.2 mg kg −1 ) at 1 h before virus infection (designated as 0 d.p.i. ), 1 d.p.i. and 2 d.p.i. obviously improved the survival rates (80%, 70% and 56%, respectively) as compared with the PBS and LNA antagomiR negative control groups (22 and 25%, respectively) ( Fig. 6a and Supplementary Fig. 6b ). These data implied that LNA antagomiR-146a could be used as a preventive agent and a therapeutic agent in the early phase of mEV71 infection. We next infected mice with mEV71 and measured miR-146a at 3 d.p.i. ; miR-146a was upregulated in mEV71-infected mice treated with LNA antagomiR negative control as compared with the mock infection. The virus-induced miR-146a was dramatically suppressed by LNA antagomiR-146a treatment at 0 and 1 d.p.i., particularly in the highly susceptible organs such as the intestine, muscle and lung ( Fig. 6b ). 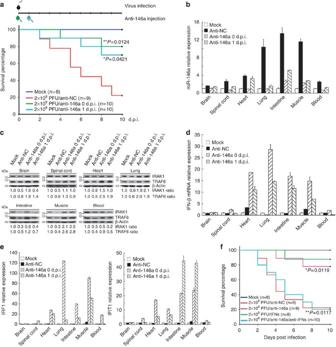Figure 6: LNA antagomiR-146a treatment improves survival and restores IFN production in EV71 mouse model. (a) LNA antagomiR-146a treatment improves survival rate. Wild-type mice were treated with LNA antagomiR-146a (1.2 mg kg−1) before or after mEV71 infection and monitored daily for survival rate. * represents the comparison between the 2 × 108PFU/anti-146a 1 d.p.i. group and the 2 × 108PFU/anti-NC group; ** represents the comparison between the 2 × 108PFU/anti-146a 0 d.p.i. group and the 2 × 108PFU/anti-NC group. (b) The increase of miR-146a expression was neutralized in EV71-infected mice by injection with LNA antagomiR-146a (n=3). (c) Suppression of IRAK1 and TRAF6 was restored by LNA antagomiR-146a injection. IFNβ (n=3) (d) and IRF1 and IFIT1 (n=3) (e) expressions were induced in EV71-infected wild-type mice injected with LNA antagomiR-146a as measured by real-time RT–PCR (mouse tissue samples pooling,n=4). (f) Anti-IFNα/β antibodies eliminated antagomiR-146a-mediated improved survival. LNA antagomiR-146a and anti-IFNα/β antibodies were sequentially injected before virus infection and the mouse survival was recorded daily. * represents the comparison between the 2 × 108PFU/anti-146a group and the 2 × 108PFU/anti-NC group; ** represents the comparison between the 2 × 108PFU/anti-146a group and the 2 × 108PFU/anti-146a/anti-IFNs group. The Kaplan–Meier method was used to estimate overall survival and the Log-rank test was performed to test the difference between survival curves. Figure 6c showed that IRAK1 and TRAF6 were restored by LNA antagomiR-146a specifically in heart, lung and muscle, and the results showed reverse correlations with the suppression of miR-146a ( Fig. 6b,c and Table 1 ). In agreement with the findings in the miR-146a −/− mouse study, IFNβ production was higher in EV71-infected wild-type mice treated with LNA antagomiR-146a at 0 and 1 d.p.i. than in the mock infection and LNA antagomiR negative control groups ( Fig. 6d and Table 1 ). The expression levels of IRF1 and IFIT1 were also detected in mice treated with LNA antagomiR-146a. These ISGs could be induced in LNA antagomiR-146a-treated mice, but not in the LNA antagomiR-NC group or mock control group ( Fig. 6e ). The percentage of paralysis, one of the signs of the CNS involvement, as well as the degree of body weight loss was significantly lower in these LNA antagomiR-146a-treated groups ( Supplementary Fig. 8b,c ). These trends are similar to the survival curve in Fig. 6a , that is, LNA antagomiR-146a not only improved the survival but also alleviated the severity of CNS involvement. To determine whether IFNs indeed play a critical role in antagomiR-146a-mediated improvement of survival, we injected mice with LNA antagomiR-146a and anti-IFNα/β antibodies sequentially before (0 d.p.i.) virus infection and recorded mouse survival daily. Fig 6f showed anti-IFNα/β antibodies almost completely eliminated the antagomiR-146a-mediated improvement in survival, and this meant that LNA antagomiR-146a improved the mouse survival through the restoration of IFNs. Figure 6: LNA antagomiR-146a treatment improves survival and restores IFN production in EV71 mouse model. ( a ) LNA antagomiR-146a treatment improves survival rate. Wild-type mice were treated with LNA antagomiR-146a (1.2 mg kg −1 ) before or after mEV71 infection and monitored daily for survival rate. * represents the comparison between the 2 × 10 8 PFU/anti-146a 1 d.p.i. group and the 2 × 10 8 PFU/anti-NC group; ** represents the comparison between the 2 × 10 8 PFU/anti-146a 0 d.p.i. group and the 2 × 10 8 PFU/anti-NC group. ( b ) The increase of miR-146a expression was neutralized in EV71-infected mice by injection with LNA antagomiR-146a ( n =3). ( c ) Suppression of IRAK1 and TRAF6 was restored by LNA antagomiR-146a injection. IFNβ ( n =3) ( d ) and IRF1 and IFIT1 ( n =3) ( e ) expressions were induced in EV71-infected wild-type mice injected with LNA antagomiR-146a as measured by real-time RT–PCR (mouse tissue samples pooling, n =4). ( f ) Anti-IFNα/β antibodies eliminated antagomiR-146a-mediated improved survival. LNA antagomiR-146a and anti-IFNα/β antibodies were sequentially injected before virus infection and the mouse survival was recorded daily. * represents the comparison between the 2 × 10 8 PFU/anti-146a group and the 2 × 10 8 PFU/anti-NC group; ** represents the comparison between the 2 × 10 8 PFU/anti-146a group and the 2 × 10 8 PFU/anti-146a/anti-IFNs group. The Kaplan–Meier method was used to estimate overall survival and the Log-rank test was performed to test the difference between survival curves. Full size image Table 1 Correlation of key components involved in the production of type I interferon in LNA antagomiR-146a-treated mice. Full size table Here we first found that enterovirus-induced AP1 promoted miR-146a expression. The miR-146a would then block the signalling for type I interferon production, and the virus could easily escape the host immune attack. A previous report showed that in human monocytic cells, LPS-mediated induction of miR-146a was NF-κB-dependent [32] . Our results suggested that EV71 infection suppressed the NF-κB signalling pathway demonstrated in RD cells, Caco-2 cells and THP-1 cells, and this discrepancy could be due to the different stimuli. The regulation between miR-146a and IRAK1 and TRAF6 also occurred in EV71 infection, and we further identified a new miR-146a BS within TRAF6 3′UTR. This new BS exhibited a synergistic effect with other identified BS on miR-146a suppressive activity [30] , [31] , [32] . To validate the effects of miR-146a in vivo , we established a mouse-adapted mEV71 from human EV71. The mice were infected with mEV71 through the natural oral route, and the clinical signs, including paralysis, loss of body weight, mortality and even pulmonary edema, were similar to those in human beings [4] , [8] , [9] , [10] , [47] , [48] , [49] , [50] , [51] . However, certain pathological observations in the EV71 infection mouse model were not clinically confirmed in human beings. In human beings, the paralysis of limbs, pulmonary edema and heart failure may be resulted from the lytic replication of EV71 in CNS while mEV71 replication can be detected in broader organs in mEV71-infected mice ( Fig. 5c ) [6] , [10] . Hence, whether the molecular pathological mechanism discovered and the new antiviral treatment developed in the EV71 infection mouse model can be applied to human beings should need to further investigate. The suppression of miR-122 by a specific LNA has been proven to attenuate HCV infection and replication in a chimpanzee model [27] as well as in a phase IIa clinical trial [55] . Thus, we introduced an LNA-based miR-146a inhibitor to demonstrate its potential application for EV71 treatment in the mEV71 infection model. Prophylactic administration of LNA antagomiR-146a or therapeutic administration in an early stage of virus infection effectively protected mEV71-infected mice from death. The application of antagomiR-146a on EV71 treatment may be limited in CNS infection due to restriction by the blood–brain barrier. Although a few reports have indicated that oligonucleotides could function in brain and silence target gene expressions in the treatment of some brain-associated diseases, it has not been established how antisense oligonucleotides cross the blood–brain barrier into the CNS [56] , [57] . Hence, the therapeutic effects of antagomiR-146a may be less evident in patients with CNS infection. For further understanding, we verified the relationships among miR-146a, IRAK1 and TRAF6, and IFN production in vivo . miR-146a induction suppressed IRAK1 and TRAF6 and further inhibited IFNβ production, while blockage of miR-146a attenuated miR-146a inhibitory activities, as demonstrated in vitro . Even though the EV71 mouse-adapted model is suitable for exploring the mechanism of pathogenesis and developing new therapeutic strategies, the limited availability of specimens in neonatal mice increases the assay difficulties. That could be why the effects of LNA antagomiR-146a were slightly different in the in vivo and in vitro models. Type I IFNs provide a first-line of defence in antiviral responses and further lead to the establishment of adaptive immunity. Administration of IFNs can limit a virus from spreading at an early phase during virus infections, while many viruses, including Influenza virus, Herpes simplex virus, Dengue virus, Marburg virus, Vesicular stomatitis virus, and foot-and-mouth disease virus [58] , [59] , [60] , [61] , [62] , [63] , [64] , [65] have evolved through several mechanisms to prevent IFN attacks by the inhibition of IFN synthesis, inactivation of secreted IFN molecules, deletion of IFNs receptors or blockage of IFN signalling. Dengue virus NS2B3 protease complex can cleave the human adaptor molecule STING, a mediator of IRF3 activation, resulting in type I IFN inhibition and augmenting the propagation of Dengue virus [64] . Marburg virus disrupts IFN production through multiple means; VP35 IID binds to double-stranded RNAs and sequestrates dsRNA from pathogen-associated molecular pattern recognition as well as inhibits the activation of interferon regulatory factor 3 (ref. 63 ). In addition, virus can escape IFN attacks by influencing or disrupting IFN signalling-associated molecules by viral components. Here we discovered a new strategy, in which a virus utilizes host factors for immune escape. Enterovirus induces cellular miR-146a expression to inhibit IFN production and escape host immune attacks, and this newly discovered mechanism is quite unlike the other known immune escape mechanisms [65] . In summary, we have identified a new virus-host interaction wherein virus infection results in AP1-mediated miR-146a induction, suppression of IRAK1 and TRAF6, and inhibition of IFN production, by which the virus escapes from host immune attacks ( Fig. 7 ). Neutralization of virus-induced miR-146a could block this signalling cascade, thereby relieving symptoms and reducing mortality. Our findings shed light on the development of a therapeutic strategy for enterovirus infections. It could be worthwhile to further investigate whether viruses other than enteroviruses also escape from host immune defence through similar mechanisms. 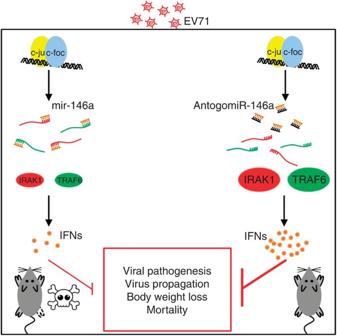Figure 7: Model for the regulatory role of miR-146a in enterovirus infection. Enterovirus-induced AP1-mediated miR-146a induction, suppression of IRAK1 and TRAF6 and inhibition of IFN production, by which virus escapes host immune attacks. Neutralization of virus-induced miR-146a by LNA antagomiR-146a can block this signalling cascade, resulting in the relief of symptoms and reduction of mortality. IFNs, interferons; IRAK1, interleukin-1 receptor-associated kinase 1; TRAF6, TNF receptor-associated factor 6. Figure 7: Model for the regulatory role of miR-146a in enterovirus infection. Enterovirus-induced AP1-mediated miR-146a induction, suppression of IRAK1 and TRAF6 and inhibition of IFN production, by which virus escapes host immune attacks. Neutralization of virus-induced miR-146a by LNA antagomiR-146a can block this signalling cascade, resulting in the relief of symptoms and reduction of mortality. IFNs, interferons; IRAK1, interleukin-1 receptor-associated kinase 1; TRAF6, TNF receptor-associated factor 6. Full size image Cell cultures and virus infection Human rhabdomyosarcoma cells line (RD) and colon adenocarcinoma cell line (Caco-2) were cultured in MEM medium with 1 mM L -glutamine, 100 units ml −1 penicillin and 100 μg ml −1 streptomycin (Life Technologies). Mediums for RD and Caco-2 cells were supplemented with 10 and 20% fetal bovine serum, respectively (Life Technologies). THP-1 cells, a kind of human monocytic cells derived from an acute monocytic leukemia patient, were cultured in RPMI-1640 medium with 5 mM L -glutamine, 100 units ml −1 penicillin, 100 μg ml −1 streptomycin and 10% fetal bovine serum. THP-1 cells were treated with PMA (phorbol-12-myristate-13-acetate) and differentiated into monocyte-derived macrophages. RD cells were used in propagation and plaque titration of PV3 (Sabin strain), CVB3 and EV71. The virus infection was performed in the serum-free condition. Aliquots of viral stocks were stored at −80 °C. All cell lines were obtained from ATCC source. RNA Extraction and miRNA profiling RNAs were extracted from virus-infected or mock-infected RD cells by Trizol reagent (Life Technologies). The expression levels of 250 human miRNAs were measured using the TaqMan MicroRNA Assays (Life Technologies). Individual real-time RT–PCR Quantification of miR-146a, Homo RNU6B, mus U6 snRNA, mus IFNβ and mus β-actin were performed using TaqMan microRNA individual assays or TaqMan gene expression assays (000468, 001093, 001973, Mm00439546_s1 and Mm00607939_s1; Life Technologies) according to the manufacturer’s instructions. In brief, real-time RT–PCR was performed using a standard protocol on an Applied Biosystems 7900HT System. The 10 μl PCR mixture included 2 μl RT product, 5 μl 2x TaqMan Universal PCR Master Mix, 0.5 μl 20x TaqMan probe and primers and 2.5 μl H 2 O. The reactions were incubated in a 96-well plate at 95 °C for 10 min, followed by 40 cycles of 95 °C for 15 s and 60 °C for 1 min. All reactions were run in triplicate. The threshold cycle is defined as the fractional cycle number at which the fluorescence passes the fixed threshold [25] . Quantification of c-jun, c-fos and TBP were performed by SYBR Green-based real-time PCR ( Supplementary Table 6 ). Western blot Cells or tissues were harvested in RIPA lysis buffer (50 mM Tris–HCl (pH 7.4), 150 mM NaCl, 1 mM EDTA, 1% Triton X-100, 0.1% SDS, 1% sodium deoxycholate, 1 mM PMSF and protease inhibitor cocktail), and the protein concentration was measured by the BCA protein assay (Bio-Rad). Proteins were resolved by 10% sodium dodecyl sulphate polyacrylamide gel electrophoresis, transferred onto PVDF membranes, blocked with 5% skimmed milk in Tris-buffered saline (20 mM Tris–HCl (pH 7.5), 150 mM NaCl and 0.5% Tween-20) and reacted with primary antibodies for β-actin (1:5,000; Sigma), Homo TRAF6 (1:200; Santa Cruz), Homo IRAK1 (1:200; Santa Cruz), c-jun (1:200; Santa Cruz), c-fos (1:200; Santa Cruz), RelA (1:500; BioLegend), Histone H3 (1:3,000; Cell Signaling), mus TRAF6 (1:200; Santa Cruz), mus IRAK1 (1:200; Santa Cruz) and V5 tag (1:5,000; Life Technologies). β-actin acted as an internal control. All original blots in the main figures are presented in Supplementary Fig. 9 . Luciferase assay All transfections were carried out in triplicate in 96-well plates. RD cells (1 × 10 4 per well) were seeded 24 h prior to transfection. The luciferase reporter constructs along with the control plasmids (pRL-TK Vector; Promega) were co-transfected into cells at the DNA ratio 5:1 in the presence of pSilencer miRNA expressing vectors (Life Technologies) as indicated by Lipofectamine LTX reagent (Life Technologies). After 48 h incubation, the Dual-Glo luciferase substrate (Promega) was added to each well and the luminescent signals were measured by Victor3 multilabel counter (PerkinElmer) according to the manufacturer's instructions. For IFNβ promoter assays, the reporter constructs were co-transfected with antagomiR-NC or antagomiR-146a into RD cells prior to virus infection. After 24 h incubation, all transfectants were infected with EV71 and assayed at indicated time points. The activity of Renilla luciferase was used as an internal control to normalize transfection efficiency. Plasmid constructions The full-length TRAF6 and IRAK1 3′UTR were amplified from complementary DNAs of RD cells by using TRAF6 luc F/TRAF6 luc R and IRAK1 luc F/IRAK1 luc R, respectively ( Supplementary Table 6 ). Paired primers (TRAF6 luc F and TRAF6 mut R1, TRAF6 mut F1 and TRAF6 luc R, TRAF6 luc F and TRAF6 mut R2, TRAF6 mut F2 and TRAF6 luc R, TRAF6 luc F and TRAF6 mut R3 and TRAF6 mut F3 and TRAF6 luc R) were used to generate the mutant-types of TRAF6 3′UTR, in which the four mutated nucleotides were underlined within the seed region of miR-146a BS by PCR-based mutagenesis method ( Supplementary Table 6 ). For mutant-types of IRAK1 3′UTR constructs, primers were designated as IRAK1 luc F, IRAK1 luc R, IRAK1 mut F1, IRAK1 mut R1, IRAK1 mut F2 and IRAK1 mut R2 ( Supplementary Table 6 ). All PCR fragments were cloned into pMIR-reporter luciferase vector (Life Technologies). The coding regions and 3′UTRs of TRAF6 and IRAK1 fragments were amplified from cDNAs of RD cells and cloned into pcDNA 3.1 expression vector (Life Technologies) along with V5 tag. The miR-146a precursor fragment was amplified by PCR-based ligation and constructed into pSilencer vector (Life Technologies) with BamHI and HindIII ( Supplementary Table 6 ). The promoter regions of miR-146a precursor and IFNβ were constructed into pGL3 basic vectors, respectively. Stable transfection of RD cells and antagomiR transfections To generate the stably TRAF6- or IRAK1-expressing cell lines, RD cells were transfected with 2 μg of plasmid DNA encoding V5-TRAF6 or V5-IRAK1 fusion protein with wild-type or mutant 3′UTR by using Lipofectamine LTX reagent (Life Technologies) and treated with G418 (1 mg ml −1 ; Life Technologies). For antagomiR transfection, trypsinized RD cells at 3 × 10 5 per ml were transfected with control antagomiR (5 pM) or specific antagomiR (5 pM) (Life Technologies) by siPORT NeoFX transfection reagent (Life Technologies) according to the manufacturer's instructions. Plaque assay EV71 plaque assays were carried out in triplicate in 6-well plates. RD cells were infected with 100 μl per well of diluted viral stocks. After 1-h incubation, the infected cells were washed and incubated for 3 days in 0.3% agarose medium overlay. Cells were fixed with formaldehyde and stained with crystal violet. Plaques were counted. JNK inhibitor treatment RD cells were seeded into 6-well plates and infected with EV71 under 20 μM JNK inhibitor (SP600125, Sigma-Aldrich), DMSO or medium only. After infection, total proteins and RNAs were extracted and assayed with western blot or real-time RT–PCR, respectively. mEV71 and LNA antagomiRs administration C57BL/6 mice were provided by the Knockout Mouse Core Laboratory of National Taiwan University Center of Genomic Medicine, housed in specific pathogen-free animal rooms, and treated according to guidelines from the National Taiwan University College of Medicine and College of Public Health Institutional Animal Care and Use Committee (IACUC). Seven-day-old male and female mice were used in this study. mEV71 was established referring to a report published by Wang, Y.F. in 2004. mEV71 was generated after four serial passages in neonate mice started from parental human EV71. Parental human EV71 was injected intraperitoneally and next generation mEV71, called 1st mEV71, was isolated from neonate mice brain tissue at 3 d.p.i. The isolated 1st mEV71 was then propagated in RD cells. The passage procedures were performed four times. To determine the 50% lethal dose (LD50), 7-day-old wild-type C57BL/6 mice were fed with indicated PFUs of mEV71. The survival of mice was monitored daily. For wild-type C57BL/6 mice and miR-146a −/− C57BL/6 mice inoculation, each group ( n =9–13) housed in the same cage was infected with indicated PFUs of mEV71 through the oral route, and the control group was fed with culture medium. The animals were monitored daily, and clinical signs, weight and mortality were recorded. All mouse tissues were obtained from scarified mice with significant clinical illness signs or at 3 d.p.i. if mice had no significant illness signs. The tissues were further assayed for real-time RT–PCR, western blot, plaque assay, immunohistochemistry staining and so on. For LNA antagomiRs injection, wild-type mice were injected with LNA antagomiR-146a (1.2 mg kg −1 ) or LNA antagomiR negative control (1.2 mg kg −1 ) through the intraperitoneal route before or after virus infection as indicated and monitored daily. The institutional animal care and use committee (IACUC) approved all animal protocols. Immunohistochemistry staining Mock-infected and virus-infected mouse sections for immunostaining were obtained from optimal cutting temperature-embedded tissues. The samples were stained with primary antibodies anti-EV71 (1:200; Millipore) at 4 °C for 12 h. The samples were washed twice with PBS, treated with goat anti-mouse IgG biotin-labeled secondary antibody (1:500; Vector Laboratories) at room temperature for 1 h and developed by ABC kit (Vector Laboratories) according to the manufacturer's instructions. The slides were then examined by microscope. Statistical analysis Student’s t- test was used to compare the miRNA expression at different time points during EV71 infection. P- value <0.05 was considered as significant and two-tailed tests were used in this study. The miRNAs with greater than twofold change of expressions at both 4 and 8 h.p.i. relative to mock infection were identified for further study. The associations of miR-146a with IRAK1 or TRAF6 and IRAK1 or TRAF6 with IFNβ are presented as coefficient of correlation ( r ) estimated by Pearson correlation method. The positive or negative r represents the positive or negative association between the two variables. How to cite this article : Ho, B.-C. et al . Inhibition of miR-146a prevents enterovirus-induced death by restoring the production of type I interferon. Nat. Commun. 5:3344 doi: 10.1038/ncomms4344 (2014).